TRPV2 is critical for the maintenance of cardiac structure and function in mice The heart has a dynamic compensatory mechanism for haemodynamic stress. However, the molecular details of how mechanical forces are transduced in the heart are unclear. Here we show that the transient receptor potential, vanilloid family type 2 (TRPV2) cation channel is critical for the maintenance of cardiac structure and function. Within 4 days of eliminating TRPV2 from hearts of the adult mice, cardiac function declines severely, with disorganization of the intercalated discs that support mechanical coupling with neighbouring myocytes and myocardial conduction defects. After 9 days, cell shortening and Ca 2+ handling by single myocytes are impaired in TRPV2-deficient hearts. TRPV2-deficient neonatal cardiomyocytes form no intercalated discs and show no extracellular Ca 2+ -dependent intracellular Ca 2+ increase and insulin-like growth factor (IGF-1) secretion in response to stretch stimulation. We further demonstrate that IGF-1 receptor/PI3K/Akt pathway signalling is significantly downregulated in TRPV2-deficient hearts, and that IGF-1 administration partially prevents chamber dilation and impairment in cardiac pump function in these hearts. Our results improve our understanding of the molecular processes underlying the maintenance of cardiac structure and function. Mechanical forces provide essential physiological information for homeostatic regulation and functional adaptation at the levels of cells and organs [1] . In cardiovascular systems, cellular mechanical responses to haemodynamic stress are crucial for normal cardiac function, and affect both the physiological and the pathological growth of the heart [2] , [3] . More specifically, an increased cardiac workload resulting from exercise, pregnancy or postnatal growth promotes the physiological growth of the heart, whereas chronic hypertension can cause pathological hypertrophy [3] . Atrophy of the heart is a complication of protracted bed rest, prolonged weightlessness during space travel, and mechanical unloading with a ventricular assist device [3] . Despite the obvious influence of mechanical load on cardiac structure and function, the molecular details of the myocardial mechanotransduction required to maintain cardiac structure and function have remained unclear. The heart is a functional syncytium composed of terminally differentiated myocytes specialized for excitation–contraction (E–C) coupling [3] . Individual cardiomyocytes are electrically and mechanically coupled at their termini, where highly organized cell–cell junctions known as intercalated discs are located [4] , [5] , [6] . The structure of intercalated discs is known to be remodelled in response to haemodynamic stress [7] . High wall stress increases the myocardial contractile force exerted as a result of cardiac hypertrophy, and the intercalated disc structure has to be optimized for physical robustness to adapt to this force [3] . By contrast, mechanical unloading causes cardiac atrophy, accompanied by disorder in the intercalated disc structure [7] , [8] , [9] , [10] . In addition, human cardiomyopathies have been associated with mutations in genes encoding components of intercalated discs, involved in mechanical coupling, and studies in mice and humans have suggested a connection between faulty myocardial mechanical coupling mechanisms and heart disease [11] , [12] , [13] , [14] , [15] . Flexibility in cardiac adaptation to haemodynamic stress probably requires the maintenance of intercalated disc structure and function by continuous monitoring of the mechanical stress at intercalated discs. Therefore, we hypothesized that cardiac mechanoreceptors at intercalated discs detect mechanical stress in the heart, maintaining myocardial structure and function in response to haemodynamic stress through the mechanical feedback system in cardiomyocytes. Members of the transient receptor potential (TRP) cation channel family are potential candidates for the mechanoreceptors responding to tension, flow or changes in cell volume [16] . Previously, we reported that recombinant TRP, vanilloid family type 2 (TRPV2) can be activated by hypotonicity- and stretch-induced mechanical stimulation in ectopic expression systems [17] , [18] . Interestingly, TRPV2 is highly localized to mammalian cardiac intercalated discs, and its increased expression at the sarcolemma is observed in dystrophic human patients and animal models deficient in dystrophin or δ-sarcoglycan [17] . To elucidate the physiological role of cardiac TRPV2, we generated temporally controlled cardiac-specific TRPV2-deficient mice. Cardiac-specific TRPV2 elimination led to a severe decline in the heart’s pump function with the disorganization of the intercalated disc structure, conduction defects and accelerated mortality. TRPV2-deficient neonatal cardiomyocytes formed no intercalated discs and showed no extracellular Ca 2+ -dependent intracellular Ca 2+ increase and IGF-1 secretion after stretch stimulation. TRPV2-deficient hearts showed downregulation of IGF-1 receptor/PI3K/Akt signalling. In addition, IGF-1 administration partially prevented chamber dilation and improved cardiac pump function in TRPV2-deficient hearts. These results suggest an indispensable role for TRPV2 in the maintenance of cardiac structure and function. Generation of cardiac-specific TRPV2-deficient mice Initially, mice carrying a TRPV2 flox/flox allele were generated by flanking exon 4 of the TRPV2 gene with two loxP sequences ( Supplementary Fig. 1 ). Excision of this segment resulted in a frameshift mutation downstream of the deletion sites. Translation from the first ATG gave rise to a short, 92 amino-acid (aa) product containing 62 aa of the original TRPV2 protein; however, most of the TRPV2 channel structure was lost after Cre -mediated recombination. We crossed mice bearing the TRPV2 flox/flox allele with a transgenic line ( MerCreMer ) expressing Cre recombinase under the control of the α-myosin heavy chain promoter in a tamoxifen-inducible cardiomyocyte-specific manner [19] to produce TRPV2 flox/flox ;MerCreMer +/− mice. To account for the deleterious effect of potential nonspecific Cre recombinase-mediated cardiotoxicity [20] , we used TRPV2 flox/+ ;MerCreMer +/− and TRPV2 flox/flox ;MerCreMer − / − littermates as age-matched controls, from which TRPV2 flox/flox ;MerCreMer +/− mice were indistinguishable in appearance. The TRPV2 flox/flox ;MerCreMer +/− mice were genotyped by PCR using primers for Cre-loxP sites and Cre recombinase ( Fig. 1a and Supplementary Fig. 1 ). In adult TRPV2 flox/flox ;MerCreMer +/− mice treated with tamoxifen for 3 days (daily dose of 8 mg kg −1 ), we confirmed successful Cre recombination by PCR amplification of cardiac genomic DNA, to detect the deleted allele ( Fig. 1b ). Consistently, the expression of TRPV2 messenger RNA was dramatically suppressed in the hearts of TRPV2-deficient mice on day 3 ( Fig. 1c ). There was an ~95% reduction in TRPV2 protein in membrane extracts of cardiac muscle from these mice after 4 days of tamoxifen treatment ( Fig. 1d ). Consistently, the TRPV2 protein was also not detectable by immunofluorescent staining at intercalated discs in the hearts of these mice, although TRPV2 was highly localized to intercalated discs in control mice ( Fig. 1e ). Hereafter, in this study, we treated TRPV2 flox/flox ;MerCreMer +/− , TRPV2 flox/+ ;MerCreMer +/− and TRPV2 flox/flox ;MerCreMer − / − mice with 8 mg kg −1 per day tamoxifen or vehicle for 4 consecutive days, then carried out analyses at different time points. 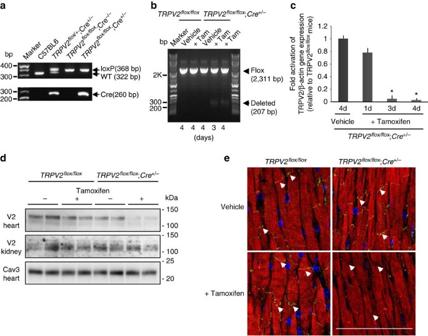Figure 1: Generation of temporally controlled cardiac-specific TRPV2-deficient mice. (a) Genotyping ofTRPV2flox/flox;MerCreMer+/−mice using tail genomic DNA. (b) Confirmation ofCrerecombination by PCR of cardiac genomic DNA. (c) TRPV2 messenger RNA expression confirmed by RT–PCR, using β-actin as an internal control gene (n=3 mice per group). Data are mean±s.e.m. *P<0.05 versus non-treated age-matchedTRPV2flox/flox;MerCreMer−/−(TRPV2flox/flox) mice. (d) Expression of TRPV2 protein in heart and kidney from tamoxifen-treated and -untreatedTRPV2flox/floxorTRPV2flox/flox;MerCreMer+/−(TRPV2flox/flox;Cre+/−) mice, using caveolin 3 as an internal control for hearts. Membrane extracts (10 μg per lane) were subjected to immunoblotting. (See full blots with marker position inSupplementary Fig. 6). (e) Triple staining of left ventricle sections with anti-TRPV2 antibody (green), phalloidin (red) and DAPI (blue). Scale bar, 100 μm. Arrows, intercalated discs. Figure 1: Generation of temporally controlled cardiac-specific TRPV2-deficient mice. ( a ) Genotyping of TRPV2 flox/flox ; MerCreMer +/− mice using tail genomic DNA. ( b ) Confirmation of Cre recombination by PCR of cardiac genomic DNA. ( c ) TRPV2 messenger RNA expression confirmed by RT–PCR, using β-actin as an internal control gene ( n =3 mice per group). Data are mean±s.e.m. * P <0.05 versus non-treated age-matched TRPV2 flox/flox ;MerCreMer −/ − ( TRPV2 flox/flox ) mice. ( d ) Expression of TRPV2 protein in heart and kidney from tamoxifen-treated and -untreated TRPV2 flox/flox or TRPV2 flox/flox ; MerCreMer +/− ( TRPV2 flox/flox ; Cre +/− ) mice, using caveolin 3 as an internal control for hearts. Membrane extracts (10 μg per lane) were subjected to immunoblotting. (See full blots with marker position in Supplementary Fig. 6 ). ( e ) Triple staining of left ventricle sections with anti-TRPV2 antibody (green), phalloidin (red) and DAPI (blue). Scale bar, 100 μm. Arrows, intercalated discs. Full size image The chamber dilation in TRPV2-deficient hearts Paraffin sections from TRPV2-deficient hearts were treated with Masson’s trichrome stain and analysed histologically. After 4 days of tamoxifen treatment, hearts from TRPV2 flox/flox ;MerCreMer +/− mice were morphologically normal with no incremental changes in the heart weight/body weight ratio or the cross-sectional area of the cardiomyocytes ( Fig. 2a–d ). However, 9 days after the onset of tamoxifen treatment, the chambers of the hearts from these mice were enlarged, as seen in the final phase of dilated cardiomyopathy ( Fig. 2a ). This dilation differed from ventricular hypertrophy as the ventricle wall was not thickened. As evidence of this, within 10 days of the onset of tamoxifen administration, the heart weight/body weight ratio and cardiomyocyte cross-sectional area in TRPV2-deficient hearts were comparable with those of control mice ( Fig. 2b,c ). In addition, the cardiomyocytes of TRPV2-deficient mice showed no cellular degeneration or intermuscular fibrosis ( Fig. 2d ). Whereas the cell–cell interfaces forming intercalated discs ran perpendicular to the muscle fibres in the hearts of TRPV2 flox/flox ;MerCreMer +/− control mice treated only with vehicle, in hearts treated with tamoxifen for 9 days, the contact areas between cells corresponding to intercalated discs were expanded, extended and irregularly shaped ( Fig. 2e ). Thus, it is possible that the chamber dilation in TRPV2-deficient hearts on day 9 was associated with cellular elongation resulting from the disorganization of the intercalated disc structure. Surprisingly, about 70% of TRPV2 flox/flox ;MerCreMer +/− mice died within 10 days of the onset of tamoxifen treatment, suggesting an indispensable role for TRPV2 in the working heart ( Fig. 2f ). 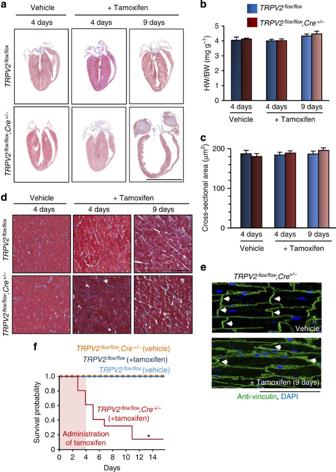Figure 2: Morphological changes and survival in TRPV2-deficient mice. TRPV2flox/flox;MerCreMer−/−(TRPV2flox/flox) andTRPV2flox/flox;MerCreMer+(TRPV2flox/flox;Cre+/−) mice, treated with tamoxifen or vehicle, were analysed on day 4 and day 9. (a) Cardiac morphology. Scale bar, 5 mm. (b) Heart weight (HW)/body weight (BW) ratio. Data are mean±s.e.m. (n=22–35 hearts per group) (c) Cross-sectional areas from paraffin sections of left ventricles. Data are mean±s.e.m. (n=122–153 cells from three hearts per group) (d) Masson’s trichrome staining of the left ventricle. Scale bar, 50 μm (e) Double staining with anti-vinculin antibody (green) and DAPI (blue). Scale bar, 100 μm. Arrowheads, intercalated discs. (f) Survival probabilities (n=55–85 per group).*P<0.05 versusTRPV2flox/flox;Cre+/−mice treated with vehicle, by log-rank tests. Figure 2: Morphological changes and survival in TRPV2-deficient mice. TRPV2 flox/flox ;MerCreMer −/ − ( TRPV2 flox/flox ) and TRPV2 flox/flox ;MerCreMer + ( TRPV2 flox/flox ;Cre +/− ) mice, treated with tamoxifen or vehicle, were analysed on day 4 and day 9. ( a ) Cardiac morphology. Scale bar, 5 mm. ( b ) Heart weight (HW)/body weight (BW) ratio. Data are mean±s.e.m. ( n =22–35 hearts per group) ( c ) Cross-sectional areas from paraffin sections of left ventricles. Data are mean±s.e.m. ( n =122–153 cells from three hearts per group) ( d ) Masson’s trichrome staining of the left ventricle. Scale bar, 50 μm ( e ) Double staining with anti-vinculin antibody (green) and DAPI (blue). Scale bar, 100 μm. Arrowheads, intercalated discs. ( f ) Survival probabilities ( n =55–85 per group). *P <0.05 versus TRPV2 flox/flox ;Cre +/− mice treated with vehicle, by log-rank tests. Full size image The cardiovascular function in TRPV2-deficient mice Echocardiography revealed a severe decline in fractional shortening and an increased left ventricular diastolic dimension 4 days after the start of tamoxifen treatment ( Fig. 3a,b ). Cardiac dysfunction was not observed in tamoxifen-treated TRPV2 flox/+ ;MerCreMer +/− mice (hetero knockout (KO) mice) for 4 days ( Supplementary Fig. 2 ). Therefore, the cardiac dysfunction seen in TRPV2-deficient mice (homo KO mice) is not due to side effects associated with the overexpression of Cre recombinase or tamoxifen administration. 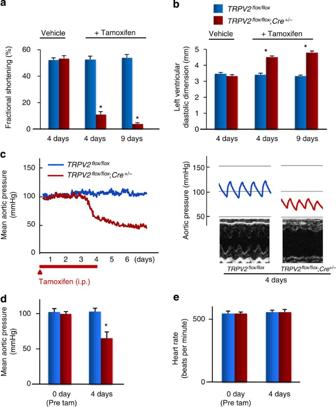Figure 3: Rapid, severe decline in cardiac pump function after TRPV2 elimination. (a,b) Echocardiographic parameters (n=5 per group). Data are means±s.e.m. *P<0.05 versusTRPV2flox/flox;Cre+/−mice treated with vehicle, by two-way analysis of variance (ANOVA) with Bonferroni’spost hoctest. (c) Representative pressure recording (left panel), and example of a pressure recording (upper right) and an echocardiograph (lower right) after tamoxifen treatment. (d,e) Mean aortic pressure and heart rate (n=3 per group). Data are means±s.e.m. *P<0.05 versus all other groups, by one-way ANOVA with Bonferroni’spost hoctest. Figure 3: Rapid, severe decline in cardiac pump function after TRPV2 elimination. ( a , b ) Echocardiographic parameters ( n =5 per group). Data are means±s.e.m. * P <0.05 versus TRPV2 flox/flox ;Cre +/− mice treated with vehicle, by two-way analysis of variance (ANOVA) with Bonferroni’s post hoc test. ( c ) Representative pressure recording (left panel), and example of a pressure recording (upper right) and an echocardiograph (lower right) after tamoxifen treatment. ( d , e ) Mean aortic pressure and heart rate ( n =3 per group). Data are means±s.e.m. * P <0.05 versus all other groups, by one-way ANOVA with Bonferroni’s post hoc test. Full size image Figure 3c,d show that aortic blood pressure also gradually dropped in TRPV2-deficient mice after 3 days of tamoxifen treatment, although the heart rate did not change ( Fig. 3e ). Notably, the time course of blood pressure decline closely paralleled the time course of Cre - loxP recombination in tamoxifen-treated TRPV2 flox/flox ;MerCreMer +/− mice ( Fig. 1b,c ).Therefore, the rapid reduction in blood pressure appeared to result from the severe decline in cardiac pump function following the elimination of TRPV2. This suggests that TRPV2 is critical for cardiac function under basal conditions. The disordered intercalated discs in TRPV2-deficient hearts Although the gross morphology of the hearts of tamoxifen-treated TRPV2 flox/flox ;MerCreMer +/− mice after 4 days was effectively normal ( Fig. 2a ), the ultrastructure of the intercalated discs was already dramatically disrupted ( Fig. 4a ), showing extensive interdigitation, irregular shapes, lacunae and widened spaces at the sites of myofibril attachment. Immunostaining for N-cadherin and β-catenin, components of adherens junctions [4] , [5] , [6] , showed a denser localization at cell–cell interfaces in TRPV2-deficient hearts compared with vehicle controls ( Fig. 4b ). The structural abnormality of intercalated disc architecture seen in TRPV2 flox/flox ; MerCreMer +/− hearts is considered synonymous with impaired mechanical interactions with neighbouring myocytes [15] . These observations suggest that the severe decline in cardiac pump function was associated with the structural disruption of intercalated discs and adherens junctions, suggesting that mechanical coupling at these sites is under the control of TRPV2. 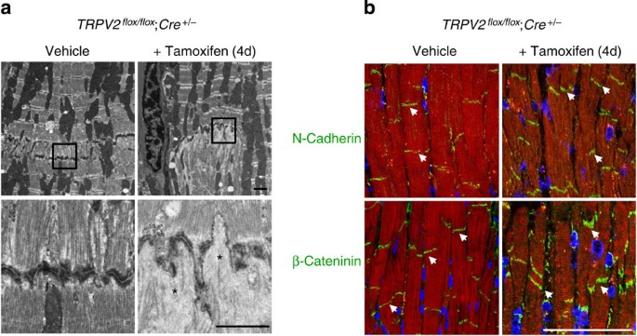Figure 4: Disorganization of intercalated discs in TRPV2-deficient hearts. (a) Electron micrographs of intercalated discs. Scale bar, 1 μm. Areas in black squares are magnified in lower panels. Asterisks, lacunae in intercalated discs. (b) Localization of N-cadherin and β-catenin in tamoxifen-treatedTRPV2flox/flox;Cre+/−mouse hearts. Scale bar, 75 μm. Arrows, intercalated discs. Figure 4: Disorganization of intercalated discs in TRPV2-deficient hearts. ( a ) Electron micrographs of intercalated discs. Scale bar, 1 μm. Areas in black squares are magnified in lower panels. Asterisks, lacunae in intercalated discs. ( b ) Localization of N-cadherin and β-catenin in tamoxifen-treated TRPV2 flox/flox ;Cre +/− mouse hearts. Scale bar, 75 μm. Arrows, intercalated discs. Full size image TRPV2 elimination affects myocardial electrical coupling A number of cardiac disorders have been described in which disruption of the intercalated disc structure significantly affects electrical coupling [4] . In TRPV2-deficient myocytes, 4 days after the onset of tamoxifen treatment, the gap junction protein connexin 43 showed diffuse localization in the intercalated discs and its expression spread along the sarcolemma over time ( Fig. 5a ). Typical electrocardiograms obtained by telemetry showed no abnormalities over the first 4 days of tamoxifen administration ( Fig. 5b ); however, after 5 days, QRS complexes time-dependently widened ( Supplementary Fig. 3 ), and 1 week after the onset of tamoxifen treatment, TRPV2-deficent hearts showed intraventricular conduction delays ( Fig. 5b ). As this phenomenon occurred several days after a drop in blood pressure was seen ( Fig. 3c ), it is likely that the disorganization of the intercalated disc architecture after the loss of TRPV2 had an indirect effect on electrical coupling with neighbouring myocytes. 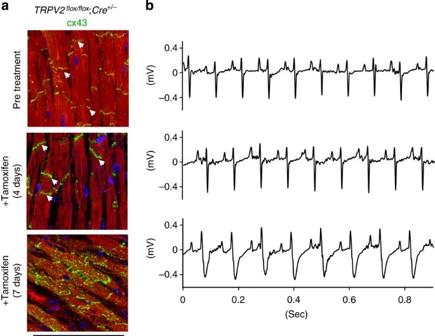Figure 5: Cardiac conduction defects after TRPV2 elimination. (a) Change in connexin 43 localization inTRPV2flox/flox;Cre+/−hearts after tamoxifen treatment. Scale bar, 100 μm. (b) Intraventricular conduction delay after TRPV2 depletion. Electrocardiographs (comparable with lead II) obtained by telemetry. Figure 5: Cardiac conduction defects after TRPV2 elimination. ( a ) Change in connexin 43 localization in TRPV2 flox/flox ;Cre +/− hearts after tamoxifen treatment. Scale bar, 100 μm. ( b ) Intraventricular conduction delay after TRPV2 depletion. Electrocardiographs (comparable with lead II) obtained by telemetry. Full size image TRPV2-deficient cardiomyocytes are fully functional Abnormal Ca 2+ handling by cardiomyocytes is a central cause of contractile dysfunction [3] . To investigate the E–C coupling of TRPV2-deficient myocytes, we analysed contractility and Ca 2+ handling in single cardiomyocytes from tamoxifen-treated and -untreated TRPV2 flox/flox ; MerCreMer +/− mice. Despite severe cardiac dysfunction, single myocytes isolated from these mice treated with tamoxifen for 4 days showed no abnormalities in cell morphology and shortening ( Fig. 6a,b ) or intracellular Ca 2+ transients evoked by electrical stimulation ( Fig. 6c ), suggesting that the ablation of TRPV2 causes no significant change in intracellular Ca 2+ handling for E–C coupling. By contrast, after 9 days of tamoxifen treatment, the isolated TRPV2-deficient cardiomyocytes showed an elongated morphology ( Fig. 6a ). These myocytes showed significantly impaired contractility ( Fig. 6b ) and Ca 2+ cycling ( Fig. 6c ), compared with vehicle-treated control cells, and electrically evoked Ca 2+ transient peaks with reduced amplitude and a slow decay speed ( Fig. 6d,e ). In addition, the Ca 2+ content of the myocyte sarcoplasmic reticulum was reduced ( Fig. 6f ), although intracellular free Ca 2+ concentrations under basal conditions were in line with the controls. 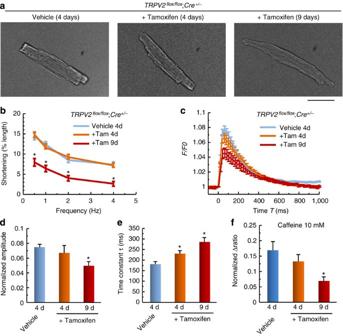Figure 6: Cardiomyocyte contractility and Ca2+handling by isolated cells from TRPV2-deficient hearts. (a) Morphology of isolated cardiomyocytes. Scale bar, 50 μm. (b) Frequency-dependent shortening of myocytes (n=100, 175, and 58 cells measured from 8, 6 and 3 hearts). (c) Indo-1 fluorescence in single cardiomyocytes stimulated at 1 Hz (n=28, 18 and 12 cells from 7, 4 and 3 hearts). (d) Peak amplitude of Ca2+transients. (e) Decay time constant obtained by fitting the decline phase. (f) Estimation of sarcoplasmic reticulum Ca2+content. Data are means±s.e.m. *P<0.05 versus vehicle control. Figure 6: Cardiomyocyte contractility and Ca 2+ handling by isolated cells from TRPV2-deficient hearts. ( a ) Morphology of isolated cardiomyocytes. Scale bar, 50 μm. ( b ) Frequency-dependent shortening of myocytes ( n =100, 175, and 58 cells measured from 8, 6 and 3 hearts). ( c ) Indo-1 fluorescence in single cardiomyocytes stimulated at 1 Hz ( n =28, 18 and 12 cells from 7, 4 and 3 hearts). ( d ) Peak amplitude of Ca 2+ transients. ( e ) Decay time constant obtained by fitting the decline phase. ( f ) Estimation of sarcoplasmic reticulum Ca 2+ content. Data are means±s.e.m. * P <0.05 versus vehicle control. Full size image The subcellular structure of cardiomyocytes and the localization of Ca 2+ regulatory proteins are well suited to their cellular functions [21] . In cardiomyocytes, Ca 2+ release for contraction occurs at distinct structures (dyads) along T-tubules, which are critical for efficient E–C coupling [22] . In the dyad space in control vehicle-treated hearts, L-type Ca 2+ channels and Na + /Ca 2+ exchangers were localized in T-tubules, and ryanodine receptors were located on sarcoplasmic reticulum membranes, so that these immunofluorescence signals appeared as well-ordered patterns ( Fig. 7a ). In TRPV2 flox/flox ;MerCreMer +/− mice treated with tamoxifen for 4 days, the key Ca 2+ regulatory proteins in cardiomyocyte E–C coupling (that is, L-type Ca 2+ channels, ryanodine receptors, and Na + /Ca 2+ exchangers) were normally expressed, and localized in T-tubules and sarcoplasmic reticulum membranes, as in vehicle controls, suggesting normal Ca 2+ handling in the cardiomyocytes ( Fig. 7a,b ). The myofilament structures were normal in these tamoxifen-treated mice for 4 days ( Fig. 7c ). Thus, the main cause of the rapid and severe decline in cardiac pump function in TRPV2-deficient hearts was not abnormal Ca 2+ handling affecting myocyte E–C coupling or disorganization of contractile filaments. 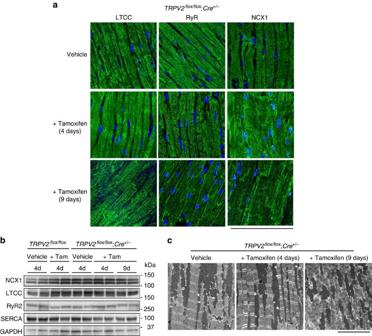Figure 7: Expression of Ca2+handling protein by isolated cardiomyocytes and electron micrographs of myofibrils in TRPV2-deficient hearts. (a) Time-dependent changes in the localization of the Ca2+regulatory proteins LTCC, RyR and NCX1 in tamoxifen-treatedTRPV2flox/flox;Cre+/−mice. Double staining with anti-LTCC antibody (green) and DAPI (blue) in cardiac muscle (left panels). Double staining with anti-RyR antibody (green) and DAPI (blue) in cardiac muscle (middle panels). Double staining with anti-NCX1 antibody (green) and DAPI (blue) in cardiomyocytes (right panels). Scale bar, 100 μm. (b) Expression of NCX1, LTCC, RyR and SERCA proteins in TRPV2-deficient heart extracts (10 μg per lane), using GAPDH as the internal control in cardiac muscle, (see full blots inSupplementary Fig. 6). (c) Electron micrographs of myofibrils in cardiomyocytes fromTRPV2flox/flox;Cre+/−mice, untreated or treated with tamoxifen. Scale bar, 5 μm. Figure 7: Expression of Ca 2+ handling protein by isolated cardiomyocytes and electron micrographs of myofibrils in TRPV2-deficient hearts. ( a ) Time-dependent changes in the localization of the Ca 2+ regulatory proteins LTCC, RyR and NCX1 in tamoxifen-treated TRPV2 flox/flox ;Cre +/− mice. Double staining with anti-LTCC antibody (green) and DAPI (blue) in cardiac muscle (left panels). Double staining with anti-RyR antibody (green) and DAPI (blue) in cardiac muscle (middle panels). Double staining with anti-NCX1 antibody (green) and DAPI (blue) in cardiomyocytes (right panels). Scale bar, 100 μm. ( b ) Expression of NCX1, LTCC, RyR and SERCA proteins in TRPV2-deficient heart extracts (10 μg per lane), using GAPDH as the internal control in cardiac muscle, (see full blots in Supplementary Fig. 6 ). ( c ) Electron micrographs of myofibrils in cardiomyocytes from TRPV2 flox/flox ;Cre +/− mice, untreated or treated with tamoxifen. Scale bar, 5 μm. Full size image Abnormal Ca 2+ handling in TRPV2-deficient myocytes In TRPV2 flox/flox ;MerCreMer +/− hearts, 9 days after the onset of tamoxifen treatment the subcellular localization of L-type Ca 2+ channels, ryanodine receptors and Na + /Ca 2+ exchangers was abnormal, representing a defect in intracellular Ca 2+ handling ( Fig. 7a ), although the levels of expression of these Ca 2+ regulatory proteins were similar to controls ( Fig. 7b ). It was possible that T-tubules and dyad structures were disordered in TRPV2-deficient hearts by day 9. In isolated cardiomyocytes at this stage, RyR activity was not only significantly lower ( Fig. 6c,d ), but the reaction area of Ca 2+ sparks elicited by electrical stimulation was also reduced and showed subcellular heterogeneity ( Supplementary Fig. 4 ). TRPV2-deficient myocytes on day 9 also showed extensive disorganization of the myofilaments needed to generate force ( Fig. 7c ). At this later stage, TRPV2-deficient myocytes showed impaired Ca 2+ handling ( Fig. 6b–f and Supplementary Fig. 4 ) and disorganization of the contractile cytoskeletal apparatus ( Fig. 7c ). Thus, eliminating TRPV2 not only led to a rapid and severe decline in normal cardiac pump function, but also resulted in a subsequent cellular dysfunction in individual myocytes. Characterization of TRPV2-deficient neonatal cardiomyocytes Intra-, inter- and extracellular mechanical forces play vital roles in the differentiation and maturation of cardiomyocytes, both in in vivo and in vitro [1] , [2] , [3] . In particular, the formation of mature intercalated discs is important during development for directing myofibrogenesis, appropriate Ca 2+ handling for E–C coupling and differentiation into synchronously beating myocytes [6] . In cultured newborn cardiomyocytes, we were able to follow the formation of intercalated discs and the reorganization of myofibrils with time in myocytes isolated by enzymatic dissociation from neonatal heart tissue [23] . When we examined the formation of intercalated discs in cultured neonatal cardiomyocytes, by staining for the gap junction protein, connexin 43, and N-cadherin ( Fig. 8a , upper and middle, first three panels), we observed that the intercalated disc structures at cell–cell interfaces showed many zigzags, sharp turns and a high degree of convolution. In control cardiomyocytes isolated from TRPV2 flox/flox ;MerCreMer −/− with or without tamoxifen treatment or TRPV2 flox/flox ;MerCreMer +/− mice cultured without tamoxifen ( Fig. 8a , all panels except for right column), we observed well-developed sarcomeres, typical localization of connexin 43 and N-cadherin to intercalated discs at cell–cell interfaces and synchronously beating myocytes. In these cardiomyocytes, NCX1 was highly expressed at the cell surface and at intercalated areas, indicating their maturation and differentiation into synchronously beating myocytes ( Fig. 8a , first three bottom panels). By contrast, TRPV2-deficient myocytes cultured with 0.2 μg ml −1 tamoxifen for 48 h formed no intercalated discs between neighbouring cells, and showed aberrant intracytoplasmic accumulation of connexin 43, internally defuse N-cadherin, and reduced expression of NCX1 ( Fig. 8a , right panels). Although we observed spontaneous weak beating in TRPV2-deficient myocytes, it was not synchronous. 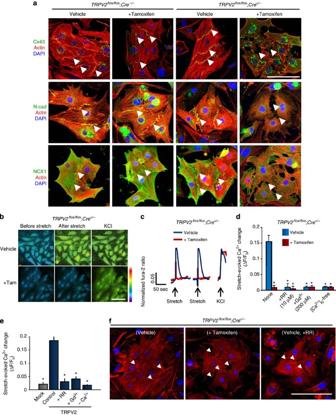Figure 8: Impairment of maturation into functional syncytia with synchronously beating cardiomyocytes in TRPV2-deficent newborn mice. (a) Isolated cardiomyocytes fromTRPV2flox/flox;Cre−/−or TRPV2flox/flox;Cre+/−newborn mice. Triple staining with anti-connexin 43 antibody (green), phalloidin (red) and DAPI (blue) in cardiomyocytes (upper panels). Triple staining with anti-N-cadherin antibody (green), phalloidin (red) and DAPI (blue) in cardiomyocytes (middle panels). Triple staining with anti-NCX1 antibody (green), phalloidin (red) and DAPI (blue) in cardiomyocytes (lower panels). Scale bar, 100 μm. (b) Fura-2-imaging of stretch-induced intracellular Ca2+dynamics in neonatal cardiomyocytes. Scale bar, 100 μm. (c) Representative trace of stretch-induced intracellular Ca2+increase. (d) Effect of mechanosensitive channel inhibitors. Data are means±s.e.m. *P<0.01 versus vehicle control (n=19–44). (e) Stretch-induced Ca2+changes in ectopically expressed TRPV2 in HEK293 cells. Data are means±s.e.m. *P<0.01 versus control. (n=23–37) (f) Isolated cardiomyocytes from newborn mice cultured with 10 μM rubidium red. Scale bar, 100 μm. Arrowheads, cell–cell junctions. Figure 8: Impairment of maturation into functional syncytia with synchronously beating cardiomyocytes in TRPV2-deficent newborn mice. ( a ) Isolated cardiomyocytes from TRPV2 flox/flox ;Cre −/− or TRPV2 flox/flox ;Cre +/− newborn mice. Triple staining with anti-connexin 43 antibody (green), phalloidin (red) and DAPI (blue) in cardiomyocytes (upper panels). Triple staining with anti-N-cadherin antibody (green), phalloidin (red) and DAPI (blue) in cardiomyocytes (middle panels). Triple staining with anti-NCX1 antibody (green), phalloidin (red) and DAPI (blue) in cardiomyocytes (lower panels). Scale bar, 100 μm. ( b ) Fura-2-imaging of stretch-induced intracellular Ca 2+ dynamics in neonatal cardiomyocytes. Scale bar, 100 μm. ( c ) Representative trace of stretch-induced intracellular Ca 2+ increase. ( d ) Effect of mechanosensitive channel inhibitors. Data are means±s.e.m. * P <0.01 versus vehicle control ( n =19–44). ( e ) Stretch-induced Ca 2+ changes in ectopically expressed TRPV2 in HEK293 cells. Data are means±s.e.m. * P <0.01 versus control. ( n =23–37) ( f ) Isolated cardiomyocytes from newborn mice cultured with 10 μM rubidium red. Scale bar, 100 μm. Arrowheads, cell–cell junctions. Full size image Previously, we reported that recombinant TRPV2 in Chinese hamster ovary cells could be activated by stretch-induced mechanical stimulation [17] , [18] . We investigated whether neonatal cardiomyocytes showed an intracellular Ca 2+ increase after stretch stimulation dependent upon TRPV2. In TRPV2 flox/flox ;MerCreMer +/− myocytes untreated with tamoxifen, an extracellular Ca 2+ -dependent intracellular Ca 2+ increase was detected after stretch stimulation, which was blocked by inhibitors of stretch-activated channels, Gd 3+ or ruthenium red (RR) ( Fig. 8b–d ). Although RR is known to block RyR, its effect is not permanent, so using a bath application should limit its effects to plasma membrane channels [24] . By contrast, no stretch-evoked Ca 2+ increase was observed in tamoxifen-treated myocytes. In addition, we confirmed the stretch-evoked Ca 2+ increase in HEK293 cells expressing TRPV2 and the blockade of this response by Gd 3+ or RR ( Fig. 8e ). These results indicate that TRPV2 is a key molecule in the stretch-induced Ca 2+ response of cardiomyocytes. Interestingly, the formation of intercalated discs and the maturation into cardiomyocytes showing the synchronized beating and alignment of myofilaments seen in vehicle-treated TRPV2 flox/flox ;MerCreMer +/− myocytes were disturbed in the presence of RR at the same level as in TRPV2-deficient myocytes ( Fig. 8f ). Taken together, these findings suggest that TRPV2 activation is required for the formation of intercalated discs connecting neighbouring myocytes and their maturation into synchronously beating myocytes. Stretch-dependent TRPV2 activation controls IGF-1 secretion Substantial evidence from genetic mouse models has demonstrated the critical role of the IGF-1 receptor/PI3K/Akt pathway in maintaining physiological cardiac morphology and function [25] . Surprisingly, the connection with neighbouring myocytes and sarcomere orientation was maintained in TRPV2-deficient myocytes, when IGF-1 was added to cultures ( Fig. 9a ). Therefore, we measured IGF-1 secretion from cardiomyocytes in culture in response to cyclic stretch stimulation at 1 Hz for 30 min. IGF-1 secretion was markedly elevated in control myocytes and was blocked by the inhibitors of stretch-activated channels, Gd 3+ or RR, whereas it was significantly reduced in TRPV2-deficient myocytes ( Fig. 9b ). 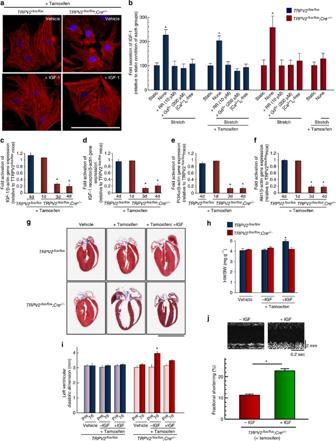Figure 9: Impairment of stretch-dependent IGF-1 secretion and IGF-1 receptor/PI3K/Akt pathway in TRPV2-deficient yocytes. (a) Isolated cardiomyocytes from newborn mice cultured with 10 μM IGF-1. Scale bar, 100 μm. (b) Stretch-dependent IGF-1 secretion by cardiomyocytes. *P<0.05 versus the other groups. Data are means±s.e.m. (c–f)IGF-1, IGF-1 receptor, PI3Kαand Aktexpression level in TRPV2-deficient hearts (n=3 mice per group). *P<0.05 versus non-treatedTRPV2flox/floxmice. Data are means±s.e.m. (g) Histological analysis 7 days after onset of IGF-1 administration and tamoxifen treatment in TRPV2-deficient mice. Scale bar, 5 mm. (h) HW/BW ratio. Data are means±s.e.m. (n=5–12 per group) *P<0.05 for tamoxifen-treatedTRPV2flox/flox;Cre+/−mice versus IGF-1-treatedTRPV2flox/flox;Cre+/−mice after 7 days. (i,j) Echocardiographic parameters (n=3 per group). (i) Data are means±s.e.m. *P<0.05 versus all the other groups. by two-way analysis of variance with Bonferroni’spost hoctest. Figure 9: Impairment of stretch-dependent IGF-1 secretion and IGF-1 receptor/PI3K/Akt pathway in TRPV2-deficient yocytes. ( a ) Isolated cardiomyocytes from newborn mice cultured with 10 μM IGF-1. Scale bar, 100 μm. ( b ) Stretch-dependent IGF-1 secretion by cardiomyocytes. * P <0.05 versus the other groups. Data are means±s.e.m. ( c – f ) IGF-1, IGF-1 receptor, PI3K α and Akt expression level in TRPV2-deficient hearts ( n =3 mice per group). * P <0.05 versus non-treated TRPV2 flox/flox mice. Data are means±s.e.m. ( g ) Histological analysis 7 days after onset of IGF-1 administration and tamoxifen treatment in TRPV2-deficient mice. Scale bar, 5 mm. ( h ) HW/BW ratio. Data are means±s.e.m. ( n =5–12 per group) * P <0.05 for tamoxifen-treated TRPV2 flox/flox ;Cre +/− mice versus IGF-1-treated TRPV2 flox/flox ;Cre +/− mice after 7 days. ( i , j ) Echocardiographic parameters ( n =3 per group). ( i ) Data are means±s.e.m. * P <0.05 versus all the other groups. by two-way analysis of variance with Bonferroni’s post hoc test. Full size image IGF-1 secreted from cardiomyocytes and fibroblast promotes the cardioprotective response to severe pressure overload by activating PI3K and its downstream effector Akt [26] , [27] . Patients with heart failure have been reported to have significantly lower IGF-1 levels compared with controls [28] . In TRPV2 flox/flox ;MerCreMer +/− mice treated with tamoxifen for 3 or 4 days, IGF-1, IGF-1 receptor, PI3K α and Akt1 expression was significantly reduced ( Fig. 9c–f ). These observations suggest that the IGF-1 receptor/PI3K/Akt pathway is downregulated in TRPV2-deficient hearts. Effects of IGF-1 administration in TRPV2-deficient hearts To investigate whether the reduced IGF-1 signalling seen in TRPV2-deficient mice represented a significant molecular basis for their observed heart failure phenotype, we treated TRPV2-deficient mice with recombinant IGF-1. In normal mice, IGF-1 administration for 1 week resulted in an increase in cardiac mass and heart-to-body weight ratio ( Fig. 9g,h ). Remarkably, in TRPV2-deficient mice, administering IGF-1 prevented both the enlargement of the left ventricular diastolic dimensions and cardiac dysfunction ( Fig. 9i,j ). In addition, expression of IGF-1 receptor, PI3K α and Akt1 were all significantly increased by the administration of IGF-1 in TRPV2-deficient hearts ( Supplementary Fig. 5 ). These results suggest that reduced IGF-1 signalling is a major factor in the heart failure observed in TRPV2-deficient mice. However, IGF-1 administration did not result in complete recovery, suggesting that other signalling pathways may also be impaired in TRPV2-deficient hearts. This study has shown a critical role for TRPV2 in the normal heart. TRPV2 is localized at intercalated discs, which are critical for detecting the mechanical forces generated by myocyte contraction. The elimination of TRPV2 from the mouse heart resulted in severe cardiac dysfunction within a few days ( Fig. 3 ), despite no impairment of myocyte contraction or E–C coupling efficiency ( Fig. 6 ). These observations suggest that the functional integration with neighbouring cardiomyocytes was weakened in TRPV2-deficient hearts. It seems that cardiomyocytes sense inadequate functional output at a cellular level and respond by increasing the number of myofibrillar attachment sites in intercalated area [7] . In a failing heart, the elevated expression of adherens junction proteins and the increase in membrane convolution and interdigitation between neighbouring cardiomyocytes seems to lead to a decrease in the flexibility of the contractile tissue and increased stiffness [7] . In TRPV2-deficient hearts, the myofilaments were disassembled at their attachment sites to intercalated discs ( Fig. 4a ). The TRPV2-deficient myocytes did not seem to sense the inadequate functional output or the severe cardiac dysfunction and therefore might have difficulty maintaining the integrity of their intercalated discs. On the other hand, cultured neonatal cardiomyocytes from TRPV2-deficient mice showed impaired formation of intercalated discs and translocation of connexin 43 and N-cadherin into cell–cell adhesion sites, and no spontaneous, synchronized beating ( Fig. 8a ). The TRPV2 inhibitor, RR, also affected intercalated disc formation in neonatal cardiomyocytes ( Fig. 8f ), implicating TRPV2 activity in the maintenance of intercalated disc integrity as well as their formation. Further experiments are needed to elucidate the molecular mechanism involved in maintaining intercalated disc structure and exactly how this function depends upon TRPV2. It is possible that TRPV2 has a pivotal role as an anchoring protein for myofibrils at intercalated discs, coordinating the transmission of mechanical forces regardless of its channel activity. The transmission of the force generated by contracting myofibrils is mediated by so-called adherens junctions, which are composed of transmembrane proteins of the cadherin family and which, in the cytoplasm, are coupled to the contracting sarcomeres by members of the catenin family [7] . Reportedly, TRPV4 associates with adherens junctions via α-catenin in the human bladder urothelium [29] . In common with several members of other TRP subfamilies [30] , the cytoplasmic region of TRPV2 is likely to couple to a rigid intracellular structural network and form ‘mechanosensitive Ca 2+ -signalosomes’ at intercalated discs. If so, eliminating TRPV2 is therefore likely to interrupt mechanical coupling with neighbouring myocytes at intercalated discs, causing severe cardiac dysfunction. In addition, we showed a significant reduction of stretch-dependent IGF-1 secretion in TRPV2-deficient myocytes ( Fig. 9b ), and a downregulation of IGF-1 receptor/PI3K/Akt signalling in TRPV2-deficient hearts ( Fig. 9c–f ). IGF-1 is continuously secreted in the normal state and in response to mechanical stress dependent on the intracellular Ca 2+ concentration [25] , [26] , [31] ; this in turn modulates myocyte PI3K signalling, which is involved in myocardial hypertrophy and heart failure [25] . It appears that the TRPV2 activation-dependent IGF-1 secretion of cardiomyocytes controls the equilibrium balance of intracellular IGF-1 receptor/PI3K/Akt signalling in response to haemodynamic stress. This forms a molecular basis for the myocyte mechanical feedback mechanism in the normal state and in response to haemodynamic stress, which is required to maintain cardiac structure and function. Therefore, loss of TRPV2 not only leads to a rapid and severe decline in normal cardiac pump function, but also triggers subsequent cellular dysfunction in individual myocytes. TRP channels are unique cellular sensors responding to a wide variety of extracellular and intracellular signals, including mechanical and osmotic stress [32] . The present study shows that TRPV2 is a candidate molecule for stretch-activated channels in myocyte intercalated discs, and is crucial for the mechanical stimulation-dependent Ca 2+ signalling of cardiomyocytes. However, it is unclear whether TRPV2 channels directly transduce mechanical stimuli or are part of a downstream signalling pathway, as discussed below. Several regulatory interactions between TRPV2 cytoplasmic domains and various signalling molecules have been investigated. Mercado et al. [33] proposed that PIP 2 is constitutively associated with the C-terminal domain of TRPV2, promoting its inhibition Ca 2+ -dependently. It is not yet certain that TRPV2 directly senses membrane lipid stretching through PIP 2 breakdown and diacylglycerol production, as has been shown for other mechanosensitive channels [34] , [35] . Therefore, to clarify the regulatory mechanism of TRPV2 activation, further electrophysiological investigations will be needed in the future. TRPV2 has been reported to translocate from an intracellular compartment to the plasma membrane in response to IGF-1 and intracellular Ca 2+ concentration [17] , [36] . Therefore, the appropriate control of these mediators might be needed for the localization of TRPV2 to the membrane in intercalated discs in working hearts. It is possible that the transmission and generation of mechanical force during contraction in response to haemodynamic stress provides the control for IGF-1 production and intracellular Ca 2+ concentrations, in which TRPV2 plays a pivotal role by continuously monitoring mechanical stress. TRPV2 activity is also directly controlled by PI3K activity, and this is independent of channel translocation to the plasma membrane [37] . Activation of PI3K by growth factors results in PIP 3 synthesis, by the phosphorylation of PIP 2 (ref. 25 ). Thus, TRPV2 activity is also likely to be regulated by the PIP 2 content, dependent on PI3K activity, and interactions with other lipids in intercalated discs. However, little is known about the lipid composition of intercalated discs. Taken together, these findings suggest that the lipid composition and potentiation of the IGF-1 receptor/PI3K/Akt signalling cascade in response to haemodynamic stress are key factors for TRPV2 activation at intercalated discs in the heart. This study has identified a molecular basis for the maintenance of cardiac structure and function, through myocyte mechanical feedback systems, in which TRPV2 plays a pivotal role ( Fig. 10 ). The integrity of intercalated discs has a large impact on force transmission and generation during muscle contraction, and is reflected in the effect of mechanical feedback on the quality of myocytes in the heart. Eliminating TRPV2 had no effect on Ca 2+ handling in myocyte E–C coupling ( Fig. 6b–f ), which is generated at dyads formed between a T-tubule and the junctional part of the sarcoplasmic reticulum. It appears that the Ca 2+ signalling involved in myocyte E–C coupling and the mechanical signal mediated by TRPV2 are spatially and temporally controlled by different signals in cardiomyocytes. Further studies might clarify the molecular mechanism of mechanotransduction mediated by TRPV2 in cardiomyocytes, and so improve our understanding of cardiac development and maturation, hypertrophic remodelling in the heart and the pathophysiology of heart disease. 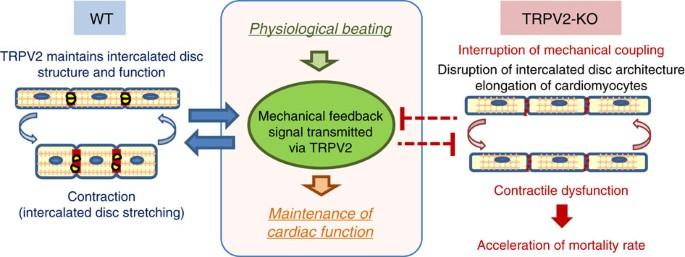Figure 10: Role of TRPV2 within the working heart. In wild-type mice, TRPV2 protein (yellow) is located in the intercalated discs (red), which is cyclically stretched and accompanied by cardiac contractions within the working heart. The mechanical feedback signal transmitted via TRPV2 is crucial for the maintenance of cardiomyocytes. TRPV2 ablation leads to the disruption of the intercalated disc architecture (red), and disorganization of sarcomere myofibril proteins at the intercalated discs (orange). These TRPV2-KO myocytes show contractile dysfunction. Therefore, the mortality rate of TRPV2-KO mice is accelerated. Thus, the mechanical feedback signal within the working heart integrates myocyte structure and function, with TRPV2 playing a pivotal role. Figure 10: Role of TRPV2 within the working heart. In wild-type mice, TRPV2 protein (yellow) is located in the intercalated discs (red), which is cyclically stretched and accompanied by cardiac contractions within the working heart. The mechanical feedback signal transmitted via TRPV2 is crucial for the maintenance of cardiomyocytes. TRPV2 ablation leads to the disruption of the intercalated disc architecture (red), and disorganization of sarcomere myofibril proteins at the intercalated discs (orange). These TRPV2-KO myocytes show contractile dysfunction. Therefore, the mortality rate of TRPV2-KO mice is accelerated. Thus, the mechanical feedback signal within the working heart integrates myocyte structure and function, with TRPV2 playing a pivotal role. Full size image Recently, Rubinstein et al. [38] reported the cardiac function of TRPV2-KO mice expressing Cre under the control of the cytomegalovirus promoter generated by Park et al [39] . They observed that cardiac function declined in TRPV2-deficient mice compared with controls, despite no histological abnormality [38] . Although there are differences in the severity of cardiac dysfunction and the depression of myocyte contractility, these results are consistent with our observations. However, the construction of their TRPV2-KO mice differed from our model in the site at which the partial elimination occurred, which corresponded to the channel pore and carboxy-terminal region of TRPV2, using a ubiquitous promoter, and the genetic background of the mice (B6129SF2/J) [39] . Park et al. [39] have reported that their model was susceptible to perinatal lethality but displayed normal thermal and mechanical nociception. They therefore suggested the possibility that compensatory mechanisms prevented the obvious phenotype of TRPV2-deficient cells being reflected in their KO mice [39] . On the other hand, the cardiac-specific elimination of TRPV2 in this study affected neither the embryonic development nor the growth after birth, in the absence of tamoxifen administration. Taken together, we believe that the acute elimination of TRPV2 function in our model might circumvent any hypothetical compensatory process. Animals Mice were housed under a 12-h light–dark cycle in a temperature-controlled environment. All the experiments were performed in male mice aged 10 weeks old (weighing 22–24 g). Littermates were used in this study to randomize genetic variation. All animal experiments were approved by the Animal Research Committee of Okayama University (Okayama, Japan), and were performed in accordance with institutional guidelines. Generation of TRPV2 conditional KO mice All experiments requiring gene recombination in this study were carried out in accordance with the institutional guideline of Okayama University (Okayama, Japan). Using cloned TRPV2 cDNA (accession code. NM011706 ) as a probe, we screened a genomic library constructed from C57/BL6J mouse DNA. The genomic clone was used to generate the targeting vector shown in Supplementary Fig. 1 , which was linearized for electroporation into C57/BL6J ES cells. After selection, G418-resistant ES clones were screened for the presence of the targeted locus by southern blot analysis. Targeted ES cells were microinjected into Balb/c mouse blastocysts, and germline transmission of the TRPV2 conditional null alleles was confirmed by southern blotting and PCR genotyping using genomic DNA extracted from mouse tail veins. We crossed mice carrying a TRPV2 flox allele with transgenic mice ( MerCreMer ) expressing tamoxifen-inducible cardiomyocyte-specific Cre recombinase to produce TRPV2 flox/flox ;MerCreMer +/− mice. Germline transmission of TRPV2 conditional null alleles was confirmed by southern blotting and PCR genotyping using the primer pair 5′-TTAAATGACTTGTGAGGGAGATAGC-3′ and 5′-CAAGTAACACAATCTACCCAAGGTC-3′, yielding 322 (wild-type) and 369 (null allele) bp products. To induce Cre -mediated recombination, we injected 10-week-old male TRPV2 flox/flox ;MerCreMer +/− , TRPV2 flox/+ ;MerCreMer +/− and TRPV2 flox/flox ;MerCreMer − / − mice intraperitoneally with 8 mg kg −1 tamoxifen (Sigma) once daily for 4 consecutive days. Tamoxifen injection and subsequent analyses were performed in a blinded fashion. Electrocardiography Transthoracic electrocardiography (ECG) was used to evaluate cardiac function with the Aplio 300 (Toshiba Medical System) and a 14-MHz transducer. The 10-week-old male mice were anesthetized initially with 2% isoflurane, and then at 1% during the examination. Left ventricular short-axis dimensions at the tip of the papillary muscles were measured on M-mode. Fractional shortening was calculated as (LVDd–LVDs)/LVDd × 100 (%). Blood pressure measurement Chronic measurements of blood pressure and ECG were performed on unrestrained, conscious mice (10-week-old, male) using a commercially available telemetry and computer-based data acquisition system (Data Sciences International) according to the manufacturer’s instructions. Briefly, a pressure-sensing catheter was implanted in the thoracic aorta via the left carotid artery, and two electrodes were placed subcutaneously on the right shoulder and left inguinal region to record lead II ECG under anaesthesia with 2% isoflurane inhalation. Mice were returned to their home cage (placed on top of telemetry receivers), and blood pressure and ECG were continuously monitored and recorded. Administration of IGF-1 Recombinant human IGF-I was purchased from Cell Science, and diluted with 0.9% NaCl at a concentration of 10 mg ml −1 and administered to mice (60 μg per day) by continuous infusion (0.25 μl h −1 ) using a mini osmotic pump (Alzert 1002). IGF-1 administration and tamoxifen treatment were started at the same time. Control mice received vehicle alone. Neonatal cardiomyocyte culture Primary cardiomyocyte cultures were prepared from ventricles of 1-day-old mice by very gentle trypsinization at room temperature, by a modification of preparation methods from rat neonatal heats [40] . Hearts were rapidly removed from neonatal TRPV2 flox/flox ;MerCreMer +/− or TRPV2 flox/flox ;MerCreMer − / − mice anesthetized with an overdose of diethyl ether. The ventricles were excised, cut into several pieces and washed three times with 10 ml ice-cold phosphate-buffered saline for 1 min by gentle shaking. The tissue pieces were digested three times with 0.06% trypsin in DMEM (8 ml) for 8 min at 37 °C by gentle agitation. The cell suspension was resuspended in DMEM with 10% fetal calf serum (FCS) to stop trypsinization, and was centrifuged at 14 g for 3 min. The cell pellets were resuspended in fresh DMEM containing 10% FCS, and plated on collagen-coated 24-well dishes at a density of 4 × 10 4 cells per well and maintained in DMEM containing 10% FCS. The formation of myocytes clusters and the spontaneous synchronized beating were confirmed by inverted microscope (CKX41, Olympus). Stretch stimulation of cardiomyocytes For stretch stimulation of cardiomyocytes, the cell suspension were plated on 1 cm 2 collagen-coated polydimethylsiloxane stretch chambers at 2 × 10 5 cells per well, and cultured. After 24 h, primary cardiomyocytes were divided into two groups and maintained for up to 2 days in DMEM containing 10% FCS, with or without tamoxifen (0.2 μM ml −1 ). Membranes were uniformly stretched by 20% for 3 s, using a computer-controlled stepping motor machine (STB-150, STREX), by a slight modification of cell-stretch culture methods [41] . One end of the chamber was firmly attached to a fixed frame, while the other was attached to a movable frame connected to a motor-driven shaft. The amplitude and frequency of stretch were controlled by a programmable microcomputer. The silicon membrane was uniformly stretched over the whole membrane area, and the lateral thinning did not exceed 1% at 20% stretch. TRPV2 deficiency did not have a discernible impact on the cardiomyocytes’ ability to adhere to the membrane, although the cell–cell interfaces with neighbouring myocytes were expanded. Stretch-induced Ca 2+ -transients in newborn cardiomyocytes Stretch-induced Ca 2+ transients were examined in cardiomyocytes loaded with 2 μM fura-2 acetoxymethyl ester (fura-2) for 30 min at 37 °C and maintained in standard Tyrode’s solution under continuous flow using a microperfusion system. Fura-2-loaded cells were alternately excited at 340 and 380 nm using a Lambda DG-4 Ultra High Speed Wavelength Switcher (Sutter Instruments) coupled to an inverted IX71 microscope with a UApo 20 × /0.75 objective lens (Olympus). Fura-2 fluorescent signals were recorded (ORCA-Flash 2.8; Hamamatsu Photonics) and analysed by a ratiometric fluorescence method using MetaFluor software (version 7.7.5.0; Molecular Devices). Isolation of adult mouse ventricular myocytes Ventricular myocytes were obtained from 10-week-old male TRPV2 flox/flox ;MerCreMer +/− and TRPV2 flox/flox ;MerCreMer − / − mice by a slight modification of Shioya’s methods [42] . Hearts were rapidly removed from adult TRPV2 flox/flox ;MerCreMer +/− or TRPV2 flox/flox ;MerCreMer − / − mice anesthetized with an overdose of pentobarbital (300 mg kg −1 , intraperitoneally), and Langendorff perfused at a constant hydrostatic pressure of 70 cm H 2 O at 37 °C using cell isolation buffer (CIB) supplemented with 0.4 mM EGTA (EGTA–CIB), which chelates calcium within the heart. CIB contained 130 mM NaCl, 5.4 mM KCl, 0.5 mM MgCl 2 , 0.33 mM NaH 2 PO 4 , 22 mM glucose, 50 nM ml −1 bovine insulin (Sigma) and 25 HEPES-NaOH (pH=7.4). Insulin was used from 1 U ml −1 stock solution in 0.1 mM HCl (pH=4.0). EGTA was from 400 mM stock in 1 M NaOH (pH=7.8). The perfusate was then switched to the enzyme solution (15 ml), which was CIB supplemented with 0.3 mM CaCl 2 , 1 mg ml −1 collagenase (Worthington Biochemical), 0.06 mg ml −1 trypsin (Sigma) and 0.06 mg ml −1 protease (Sigma). Once the tissue had undergone complete digestion, the ventricles were excised, cut into several pieces and further digested in fresh enzyme solution (15 ml) for 15–20 min at 37 °C until they were mostly dissociated. In this enzyme solution, the CaCl 2 level was increased to 0.7 mM, and 2 mg ml −1 BSA (Sigma) was supplemented. The cell suspension was centrifuged at 14 g for 3 min. The cell pellet (~0.1 ml) was resuspended in CIB supplemented with 1.2 mM CaCl 2 and 2 mg ml −1 BSA, and then incubated at 37 °C for 10 min, centrifuged (14 g , 3 min) and resuspended in 10 ml Tyroad solution supplemented with 2 mg ml −1 BSA. Tyrode’s solution contained 140 mM NaCl, 5.4 mM KCl, 1.8 mM CaCl 2 , 0.5 mM MgCl 2 , 0.33 mM NaH 2 PO 4 , 11 mM glucose and 5 mM HEPES-NaOH (pH=7.4) [40] , [42] . Cell shortening and Ca 2+ transients in adult cardiomyocytes Isolated cardiomyocytes were loaded with 10 μmol l −1 Indo-1 AM (Invitrogen) and electrically stimulated at 1 Hz using a two-platinum electrode insert connected to a bipolar stimulator (Nihon Kohden, SEN-3301) on the stage of an inverted microscope (IX71, Olympus) with a × 20 water immersion objective lens (UApo N340, Olympus). Calcium transients were measured as the ratio of fluorescence emitted at 405/480 nm after excitation at 340 nm using a high-performance Evolve EMCCD camera (Photometrics). Cardiomyocytes were maintained under continuous flow in standard Tyrode’s solution, exchanged using a microperfusion system. For measuring caffeine-induced calcium transients, cells were paced at 1 Hz prior to induction of caffeine contractures. Electrical stimulation was stopped 15 s before rapid perfusion with a 10 mmol l −1 caffeine solution. The experiments were recorded and analysed using MetaMorph software (version 7.7.1.0; Molecular Devices). Results were the means of the fluorescent signals from 10–20 cardiomyocytes from a single heart. Measure of IGF-1 concentration IGF-1 concentrations were measured in conditioned media from stretched and unstretched myocytes in a sandwich ELISA using mouse standards, according to the manufacturer’s guidelines (R&D Systems), which quotes the sensitivity of this assay as 30 ng ml −1 . Standard curves and positive controls were included in each assay, and IGF-1 concentrations were obtained by interpolation. Real-time PCR The Mouse PI3K-AKT Signalling Pathway RT 2 Profiler PCR Array was purchased from Qiagen. Total RNA extracted from TRPV2 flox/flox ;MerCreMer +/− or TRPV2 flox/flox ;MerCreMer − / − hearts with or without tamoxifen were reverse transcribed into cDNA with oligo (dT) primers using Superpscript III. Real-time PCR was performed with Step-One plus TM (Applied Biosystem). Statistical analysis of the results was performed with the Δ C t value ( C t gene of interest − C t β-actin ). Relative gene expression was obtained using the ΔΔ C t method ( C t sample − C t calibrator ) using the TRPV2 flox/flox ;MerCreMer − / − hearts without tamoxifen as a calibrator. Histology Hearts were excised and immediately fixed in buffered 4% paraformaldehyde, embedded in paraffin and sectioned to a thickness of 4 μm. We stained serial sections of samples with Masson’s trichrome to evaluate gross morphology and fibrosis. The preparations were examined under a light microscope (SZX7 or BX43, Olympus). Electron microscopy For electron microscopy, excised hearts were fixed in 2% paraformaldehyde/2% glutaraldehyde in 0.1 M phosphate buffer, postfixed with 2% OsO4 in 0.1 M phosphate buffer and stained with uranyl acetate and lead citrate. The microtome sections were examined under a JEM-1200 electron microscope (Nihondensi Co., Japan). Antibodies The following antibodies were used for immunostaining or immunoblot analysis: anti-TRPV2 (1:200 dilution, AB5398, Millipore); anti-vinculin (1:100 dilution, V9131, Sigma); anti-connexin 43 (1:100 dilution, C6219, Sigma); anti-N-cadherin (1:100 dilution, 3B9, life technologies); anti-Cav3 (1:1,000 dilution, 610420, BD Pharmingen,); anti-LTCC (1:1,000 dilution, ACC033, Alomone); anti-SERCA (1:1,000 dilution, MA3919, Thermo); and anti-RyR (1:1,000 dilution, MA3916, Thermo). The anti-NCX antibody was generated in our laboratory (1:1,000 dilution). Immunocytochemistry For immunocytochemistry, 5 μm frozen heart sections embedded in OCT compound (Tissue-Tek) were permeabilized with 0.1% Triton X-100 and incubated with primary antibodies. For immunostaining of rat cardiomyocytes, cells immobilized on collagen-coated glass slides were fixed with 4% paraformaldehyde for 15 min at room temperature, permeabilized with 0.1% Triton X-100 and then stained with primary antibodies.These samples were then treated with Alexa Flour 488-conjugated anti-rabbit IgG (A11008, Life Technologies) or Alexa Flour 488-conjugated anti-mouse IgG (A11001, Life Technologies). Cells or secrions were examined using a confocal microscope (Fluoview FV1000, Olympus) mounted on an Olympus IX81 epifluorescence microscope with a UPlanSApo × 60/1.35 oil immersion objective lens (Olympus). Immunoblotting Mice hearts and kidneys were homogenized in a Hiscotron homogenizer (NITI-ON) in lysis buffer containing 20 mM HEPES (pH 7.4), 150 mM NaCl, 1% sodium deoxycholate, 1% SDS, 2 μg ml −1 leupeptin, 1 μg ml −1 aprotinin, 200 μM phenylmethylsulfonyl fluoride, and 200 μM benzamidine hydrochloride. The lysates were centrifuged at 100,000 g for 20 min and the supernatants were used for immunoblot analysis. Immunoreactive bands were visualized using a chemiluminescence detection system (Perkin Elmer) and an LAS3000 Luminescent Image Analyzer (Fuji Film). Data analysis Data were analysed by individuals who were blinded to the genotype, drug treatment or operation. Data presented here were reproducible in at least three independent experiments. Results are shown as the mean±s.e.m. Paired data were evaluated using a Student’s t -test. Two-way analysis of variance with Bonferroni’s post hoc test was used for multiple comparisons wherever appropriate. The Kaplan–Meier method with a log-rank test was used for survival analysis. P <0.05 was considered statistically significant. How to cite this article : Katanosaka, Y. et al. TRPV2 is critical for the maintenance of cardiac structure and function in mice. Nat. Commun. 5:3932 doi: 10.1038/ncomms4932 (2014).